Structure and mechanism of an intramembrane liponucleotide synthetase central for phospholipid biosynthesis Phospholipids are elemental building-block molecules for biological membranes. Biosynthesis of phosphatidylinositol, phosphatidylglycerol and phosphatidylserine requires a central liponucleotide intermediate named cytidine-diphosphate diacylglycerol (CDP-DAG). The CDP-DAG synthetase (Cds) is an integral membrane enzyme catalysing the formation of CDP-DAG, an essential step for phosphoinositide recycling during signal transduction. Here we report the structure of the Cds from Thermotoga maritima (TmCdsA) at 3.4 Å resolution. TmCdsA forms a homodimer and each monomer contains nine transmembrane helices arranged into a novel fold with three domains. An unusual funnel-shaped cavity penetrates half way into the membrane, allowing the enzyme to simultaneously accept hydrophilic substrate (cytidine 5′-triphosphate (CTP)/deoxy-CTP) from cytoplasm and hydrophobic substrate (phosphatidic acid) from membrane. Located at the bottom of the cavity, a Mg 2+ -K + hetero-di-metal centre coordinated by an Asp-Asp dyad serves as the cofactor of TmCdsA. The results suggest a two-metal-ion catalytic mechanism for the Cds-mediated synthesis of CDP-DAG at the membrane–cytoplasm interface. Glycerophosphate-based phospholipids are the major components of biological membranes, including the plasma membrane and organelle membranes. Several different glycerophospholipid species with diverse head groups exist in various biological membranes, including phosphatidylglycerol (PG), cardiolipin, phosphatidylcholine, phosphatidylethanolamine, phosphatidylinositol (PI), phosphatidylserine (PS) and phosphatidic acid (PA). The physical and chemical properties of the phospholipids are fundamental to the formation and stability of bilayer membranes that can serve as permeability barriers to hydrophilic substances (such as ions and metabolites) [1] . This is not only essential to the establishment of transmembrane electrochemical potentials in bioenergetic processes, but also supports all kinds of intracellular activities highly dependent on the compartmentation of intracellular spaces. Besides, the phospholipid bilayers also provide compatible environments for the biogenesis and metabolism of amphipathic biological molecules including lipids and membrane proteins [2] , [3] , [4] , [5] . Moreover, the phosphorylated derivatives of PI (phosphoinositides) are important regulatory molecules functioning in cell signalling and membrane trafficking [6] , [7] , and PS is involved in apoptosis and immune regulation [8] . In 1960s, Kennedy and co-workers discovered that a liponucleotide, named cytidine-diphosphate diacylglycerol (also known as CDP-DAG), is a key precursor for the biosynthesis of PI [9] , PG [10] , [11] and PS [12] . The early works also demonstrated that CDP-DAG is at the branch point of diverse biochemical pathways leading to the synthesis of phospholipids with various head groups [13] , [14] . The CDP-DAG-mediated pathways are pivotal sources for the de novo synthesis of phospholipids in both prokaryotes and eukaryotes ( Supplementary Fig. 1 ). It was found that CDP-DAG is produced through enzymatic synthesis from cytidine 5′-triphosphate (CTP) and PA, whereas a molecule of pyrophosphate is released as a by-product of the reaction [15] , [16] ( Fig. 1a,b ). The gene encoding Escherichia coli CDP-DAG synthetase (Cds, EC 2.7.7.41) was cloned [17] , and the protein was purified and characterized as a membrane-bound enzyme with strict selection for CTP or deoxy-CTP (dCTP) against other nucleotides [18] . The enzyme adopts a sequential reaction mechanism [18] , [19] and exhibits a preference for PAs with at least one double bond on either of their fatty acyl chains [18] . Later, a eukaryotic Cds was purified from Saccharomyces cerevisiae [20] and the CDS1 gene encoding it was found to be essential for yeast cell growth [21] . Molecular genetic studies on the Cds mutants of Drosophila and zebra fish revealed that Cds has a central role in phototransduction [22] and vascular morphogenesis [23] by controlling the availability of phosphoinositide 4,5 biphosphate through the phosphoinositide-recycling pathway ( Supplementary Fig. 1b ). In mouse and human, two homologous genes of Cds ( CDS1 and CDS2 ) were cloned and exhibited distinct expression pattern in different tissues [24] , [25] , [26] , [27] . For plants and cyanobacteria, knockout of Cds homologues impaired the biosynthesis of PG, an essential lipid for the proper functioning of photosynthesis [28] , [29] . Despite the central role of Cds in phospholipid biosynthesis and its important physiological functions, little is known about the architecture of its active site or the structural bases for the intramembrane enzyme to selectively bind and convert two substrate molecules with distinct properties and from different cellular milieus. 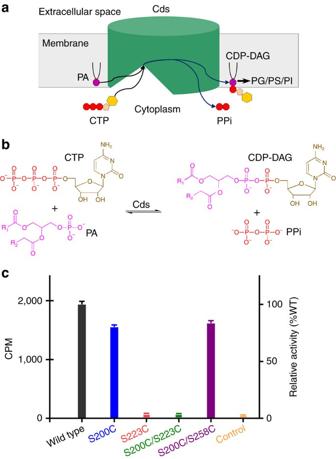Figure 1: The fundamental role of Cds enzyme in phospholipid biosynthesis. (a) A cartoon model illustrating the functional role of the membrane-embedded Cds enzyme in phospholipid biosynthesis. PA, phosphatidic acid; PG, phosphatidylglycerol; PS, phosphatidylserine; PI, phosphatidylinositol. (b) The chemical reaction of CDP-DAG synthesis catalysed by Cds. (c) The activities of wild-type TmCdsA and the cysteine mutants (S200C, S223C, S200C/S223C and S200C/S258C) in synthesizing3H-labelled CDP-DAG product. CPM, count per minute of the radioactivity measured for the hydrophobic products extracted in the organic phase. The control is the parallel reaction set up without enzyme added. The error bars denote the standard error of the mean (s.e.m.,n=4 except for S200C which hasn=3 instead). Figure 1: The fundamental role of Cds enzyme in phospholipid biosynthesis. ( a ) A cartoon model illustrating the functional role of the membrane-embedded Cds enzyme in phospholipid biosynthesis. PA, phosphatidic acid; PG, phosphatidylglycerol; PS, phosphatidylserine; PI, phosphatidylinositol. ( b ) The chemical reaction of CDP-DAG synthesis catalysed by Cds. ( c ) The activities of wild-type TmCdsA and the cysteine mutants (S200C, S223C, S200C/S223C and S200C/S258C) in synthesizing 3 H-labelled CDP-DAG product. CPM, count per minute of the radioactivity measured for the hydrophobic products extracted in the organic phase. The control is the parallel reaction set up without enzyme added. The error bars denote the standard error of the mean (s.e.m., n =4 except for S200C which has n =3 instead). Full size image Overall structure For structural studies on the Cds family, a double-cysteine mutant (S200C/S223C) of the Cds homologue from T. maritima (TmCdsA) is crystallized readily along with methylmercury chloride. With improved conformational homogeneity of this double-cysteine mutant protein and the mercury-stabilized crystal contact sites involving the engineered Cys200 residues ( Supplementary Fig. 2 ), the diffraction limits of the TmCdsA crystals have been dramatically improved from ~7 to 3.4 Å resolution. The refined structure contains around 98% of TmCdsA polypeptide chains with good statistics and geometric features ( Table 1 ), and fits well with the electron densities ( Fig. 2 ). The accuracy of sequence registration in the structure is verified by 11 site-specific mercury labels bound to the endogenous and engineered Cys residues ( Supplementary Fig. 3c,d ). Table 1 Data collection, phasing and refinement statistics for TmCdsA structures. 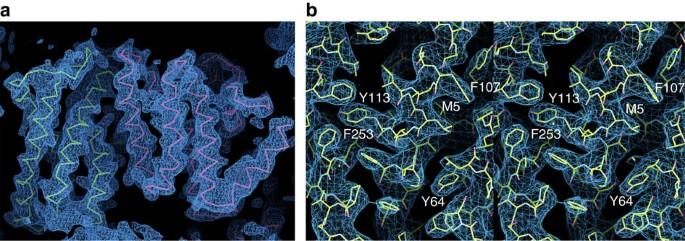Figure 2: Electron density maps of TmCdsA. (a) 2Fo−Fcmap (contoured at 1.2 × σ level) of the TmCdsA structure refined at 3.4 Å resolution and viewed along the membrane plane. (b) A zoom-in stereo view of the 2Fo-Fcmap (contoured at 1.2 × σ level) at the transmembrane region with stick models superposed on the map. Full size table Figure 2: Electron density maps of TmCdsA. ( a ) 2 F o − F c map (contoured at 1.2 × σ level) of the TmCdsA structure refined at 3.4 Å resolution and viewed along the membrane plane. ( b ) A zoom-in stereo view of the 2 F o - F c map (contoured at 1.2 × σ level) at the transmembrane region with stick models superposed on the map. Full size image The S200C/S223C mutant is inactive and its overall structure closely resembles that of an active mutant (S200C/S258C), which maintains 83.6% of wild-type activity ( Fig. 1c and Supplementary Fig. 4 ). Mutation of Ser200 to Cys only has minor effect on the enzyme activity, whereas the S223C mutation nearly abolishes the activity ( Fig. 1c ). Between the two structures, there are some subtle deviations at the N-terminal region and the two long cytoplasmic loops, reflecting the flexibility of these regions ( Supplementary Fig. 4c ). The S223C mutation enhances the interactions between the A-loop and M8 helix and reduces their flexibility, which is apparently related to the loss of activity. On the other hand, because the S223C mutation stabilizes the A-loop region that is involved in crystal packing ( Supplementary Fig. 2c ), the S200C/S223C mutant crystallizes more reproducibly than the S200C/S258C mutant. Nevertheless, both the structures represent the conformational state of TmCdsA in the substrate-free form. As they are very similar at this state, the structure of S200C/S223C is used for further analysis and characterization. The asymmetric unit contains an arch-shaped homodimer with a pseudo- C 2 axis running through the monomer–monomer interface ( Fig. 3a,b ). About 3980-Å 2 surface area is buried upon dimerization, indicating the dimeric form is a stable oligomeric state of TmCdsA. Crosslinking and multi-angle light-scattering experiments further confirm that TmCdsA is also a dimer in solution ( Supplementary Fig. 5 ). The two monomers superpose with root mean square deviation of α-carbon at 0.29 Å, suggesting they are nearly identical in overall structure. Each TmCdsA monomer contains nine transmembrane helices, namely M1–9 helices as shown in Fig. 3c,d . The M1, 3, 4, 5, 8 and 9 helices all bear small bending-angle (15–40°) kinks around proline residues, whereas M9 has one additional large-angle kink (~65°) around Gly250 ( Fig. 3d ). The C-terminus of TmCdsA is located at the periplasmic side according to the previous topology analysis result [30] . The N-terminus is thereby positioned on the cytoplasmic side considering that an odd number of transmembrane helices are observed. As shown in Fig. 3c,d , the TmCdsA monomer is organized into three individual domains appearing like the petals of a flower. They are named the N-terminal domain (NTD, containing M1 helix), the middle domain (containing M2–5 helices) at the dimerization interface and the C-terminal domain (CTD, containing M6–9 helices). Sequence alignment of various prokaryotic Cds homologues indicates that the CTD has the highest degree of conservation, whereas the NTD is moderately conserved and the middle domain is the least conserved among them ( Supplementary Fig. 6 ). 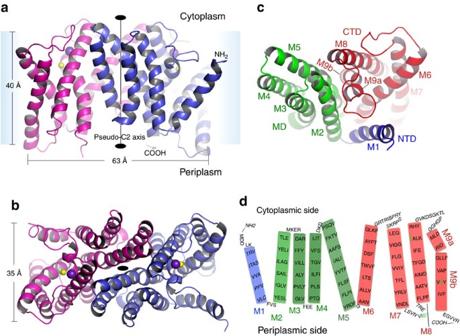Figure 3: The overall structure of TmCdsA. (a,b) TmCdsA dimer viewed along the membrane plane (a) and along the membrane normal from cytoplasmic side (b), respectively. The protein backbone of the S200C/S223C mutant is shown as cartoon models and the Mg2+/K+ions are shown as yellow/purple sphere models. The blue shades indicate the approximate location of the membrane. The monomer in blue (residues 4–270) is traced five residues longer at the N-terminal region than the monomer in magenta (residues 9–270). (c) Structure of a TmCdsA monomer with each individual domain coloured in blue, green or red. CTD, C-terminal domain; MD, middle domain;NTD, N-terminal domain . (d) Topological organization of the transmembrane helices within TmCdsA. The green ‘S’ characters labelled by * symbol indicate the location of S200, S223 and S258 residues, which are mutated into cysteine residues for crystallization purpose in this study. Figure 3: The overall structure of TmCdsA. ( a , b ) TmCdsA dimer viewed along the membrane plane ( a ) and along the membrane normal from cytoplasmic side ( b ), respectively. The protein backbone of the S200C/S223C mutant is shown as cartoon models and the Mg 2+ /K + ions are shown as yellow/purple sphere models. The blue shades indicate the approximate location of the membrane. The monomer in blue (residues 4–270) is traced five residues longer at the N-terminal region than the monomer in magenta (residues 9–270). ( c ) Structure of a TmCdsA monomer with each individual domain coloured in blue, green or red. CTD, C-terminal domain; MD, middle domain;NTD, N-terminal domain . ( d ) Topological organization of the transmembrane helices within TmCdsA. The green ‘S’ characters labelled by * symbol indicate the location of S200, S223 and S258 residues, which are mutated into cysteine residues for crystallization purpose in this study. Full size image Locations of the metal-ion cofactors Previous biochemical studies demonstrated that both prokaryotic and eukaryotic Cds enzymes require the presence of Mg 2+ ion for their activities [15] , [18] , [19] , [20] , [31] , [32] , whereas K + ion at 25–200 mM concentration stimulated the activity of M. smegmatis CdsA by ~30-fold in comparison to the enzyme with Mg 2+ alone [31] . As shown in Fig. 4a,b , the activity of TmCdsA reaches the highest level in the presence of 2 mM Mg 2+ and 50–200 mM K + . When there is only K + ion included in the reaction, the activity of TmCdsA is abolished in the absence of Mg 2+ ( Fig. 4b , dark curve), demonstrating the absolute requirement of Mg 2+ ion for TmCdsA activity. When [Mg 2+ ] is gradually increased in the reactions ( Fig. 4a ), the enzyme activity rises to the highest level at around 2 mM concentration. 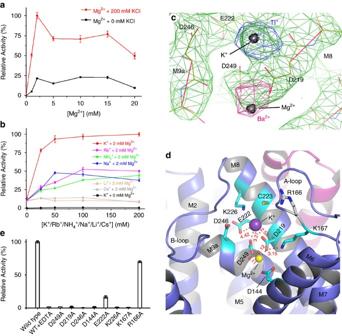Figure 4: Architecture of the active site of TmCdsA. (a) Mg2+-dependent activity changes of TmCdsA with or without 200 mM KCl. The error bars indicate s.e.m. andn=3 for the data points with [Mg2+]=2 or 10 mM (+0 or 200 mM KCl), whereas the others are withn=4. (b) The effect of increasing monovalent cation (K+, Rb+, NH4+, Na+, Li+or Cs+) concentration on the activity of TmCdsA. The lowest dark curve is measured with variable K+concentration and in the absence of Mg2+ion, whereas the other curves are measured in the presence of 2 mM Mg2+and variable concentrations of different monovalent cations.n=3 for the following data points measured with 2 mM Mg2+: [K+]=50, 200 mM; [Na+]=200 mM; [NH4+]=0 mM; [Li+]=0, 200 mM; [Cs+]=0, 25, 50 mM; [Rb+]=0, 50 mM.n=4 for the others. (c) Isomorphous difference Fourier peaks of theFBa−FMg(4.5 Å, magenta) andFTl−FK(4.5 Å, blue) maps contoured at +8.0 × σ level. Green mesh is the 3.4 Å-resolution 2Fo−Fcmap (contoured at +2.0 × σ level) of the crystal containing both Mg2+and K+ions. The Mg2+and K+ions are shown as silver bullets. The peak of Ba2+ion deviates slightly from the positions of Mg2+site because of minor changes in the unit cell dimensions of the Ba2+-soaked crystal. (d) The key amino-acid residues surrounding the Mg2+-K+di-metal centre in TmCdsA. (e) Mutagenesis analyses on the functional role of the charged residues around the di-metal centre. The activity of the wild-type enzyme was normalized as 100% relative activity after being subtracted with the negative control data (parallel reactions without enzyme added), whereas those of mutants and WT+EDTA are presented as relative percentage activity in comparison to the wild-type enzyme. The error bars denote s.e.m.,n=3 for the wild type, D249A, D219A, D246A and K167A, orn=4 for WT+EDTA, D144A, E222A, K226A and R166A. Figure 4: Architecture of the active site of TmCdsA. ( a ) Mg 2+ -dependent activity changes of TmCdsA with or without 200 mM KCl. The error bars indicate s.e.m. and n =3 for the data points with [Mg 2+ ]=2 or 10 mM (+0 or 200 mM KCl), whereas the others are with n =4. ( b ) The effect of increasing monovalent cation (K + , Rb + , NH 4 + , Na + , Li + or Cs + ) concentration on the activity of TmCdsA. The lowest dark curve is measured with variable K + concentration and in the absence of Mg 2+ ion, whereas the other curves are measured in the presence of 2 mM Mg 2+ and variable concentrations of different monovalent cations. n =3 for the following data points measured with 2 mM Mg 2+ : [K + ]=50, 200 mM; [Na + ]=200 mM; [NH 4 + ]=0 mM; [Li + ]=0, 200 mM; [Cs + ]=0, 25, 50 mM; [Rb + ]=0, 50 mM. n =4 for the others. ( c ) Isomorphous difference Fourier peaks of the F Ba − F Mg (4.5 Å, magenta) and F Tl − F K (4.5 Å, blue) maps contoured at +8.0 × σ level. Green mesh is the 3.4 Å-resolution 2 F o − F c map (contoured at +2.0 × σ level) of the crystal containing both Mg 2+ and K + ions. The Mg 2+ and K + ions are shown as silver bullets. The peak of Ba 2+ ion deviates slightly from the positions of Mg 2+ site because of minor changes in the unit cell dimensions of the Ba 2+ -soaked crystal. ( d ) The key amino-acid residues surrounding the Mg 2+ -K + di-metal centre in TmCdsA. ( e ) Mutagenesis analyses on the functional role of the charged residues around the di-metal centre. The activity of the wild-type enzyme was normalized as 100% relative activity after being subtracted with the negative control data (parallel reactions without enzyme added), whereas those of mutants and WT+EDTA are presented as relative percentage activity in comparison to the wild-type enzyme. The error bars denote s.e.m., n =3 for the wild type, D249A, D219A, D246A and K167A, or n =4 for WT+EDTA, D144A, E222A, K226A and R166A. Full size image When there is no monovalent cation added to the reactions, TmCdsA can merely reach 10–23% of its best activity at 2–20 mM Mg 2+ ( Fig. 4a , dark curve). Upon titrating K + ion into the reactions with 2 mM Mg 2+ added, the activity has a steep rise and reaches a plateau at [K + ] above 50 mM ( Fig. 4b , red curve). Among the six different monovalent cations (K + /Rb + /NH 4 + /Na + /Li + /Cs + ) tested, only K + ion can support the maximal stimulation on the enzyme activity. Na + , Rb + or NH 4 + ions can also stimulate TmCdsA activity, but to a lower level when compared with the effect of K + ion ( Fig. 4b , blue, purple and green curves). Li + or Cs + ions barely have any stimulatory effect on TmCdsA activity ( Fig. 4b , golden and grey curves). The large contrasts between the effect of K + and those of Li + /Cs + ions (up to tenfold difference at 200 mM) demonstrate that the stimulation of enzyme activity by K + ion is not due to the general effect of increasing ionic strength on protein stability but is a specific effect originating from the selective recognition of K + ion at the active site of TmCdsA. As K + ion is the dominating intracellular monovalent cation, the effect of K + ion is more physiologically relevant than those of other monovalent cations. All these results collectively prove that Mg 2+ and K + ions are both essential for TmCdsA to achieve its maximal activity and they are irreplaceable for each other in the catalytic function of TmCdsA. The data also suggest that TmCdsA contains two individual selective cation-binding sites within or around its active site. To reveal the binding sites for Mg 2+ and K + ions within TmCdsA and identify the amino-acid residues responsible for coordinating these two distinct cations, we have prepared BaCl 2 -, MnCl 2 -, TlNO 3 - or CsCl-soaked crystals to probe the binding sites of divalent and monovalent cations in TmCdsA. The Ba 2+ /Mn 2+ and Tl + /Cs + ions are used as heavy ionic surrogates for the detection of Mg 2+ and K + ion-binding sites, respectively. The F Ba − F Mg isomorphous difference Fourier map exhibits a single strong Ba 2+ peak between Asp219 and Asp249 ( Fig. 4c ), whereas the F Tl − F K difference map shows a strong Tl + peak at a different position above the Ba 2+ peak ( Fig. 4c ). The anomalous difference Fourier maps further confirm the existence of specific and distinct binding sites for Ba 2+ and Tl + ions in TmCdsA ( Supplementary Fig. 7a ). Moreover, the Mn 2+ - or Cs + -soaked crystals exhibit strong isomorphous and anomalous difference Fourier peaks around the corresponding positions where Ba 2+ or Tl + binds ( Supplementary Fig. 7b ). Thus, it is evident that the lower site is specific for divalent cation binding, whereas the upper site selects monovalent cation. The two binding sites can be occupied simultaneously by monovalent and divalent cations, respectively, as indicated by the isomorphous and anomalous difference Fourier maps of a crystal soaked in the solution containing both Rb + and Mn 2+ ions ( Supplementary Fig. 8 ). For the structure solved with a crystal containing 25 mM MgCl 2 and 100 mM KCl, the two distinct cation-binding sites capable of accepting Ba 2+ /Mn 2+ and Tl + /Cs + /Rb + ions are thereby assigned as Mg 2+ - and K + -binding sites, respectively ( Fig. 4d ). Near the central region of CTD from each TmCdsA monomer, the Mg 2+ ion is coordinated, at distances of 2.1 Å, by the carboxyl groups of two Asp residues, namely Asp219 and Asp249 ( Fig. 4d ). This binding site is located around the glycine-kink region between M9a and M9b helices. In the meantime, the K + ion is positioned 5.9 Å from the Mg 2+ -binding site and is coordinated by the carboxyl group of Asp219 at a distance of 2.5 Å. The closest distance between the carboxyl groups of Glu222/Asp249 and K + ion is 4.4/3.3 Å, suggesting they also contribute to the binding of K + ion. Architecture of the active site To further dissect the functional roles of the charged amino-acid residues surrounding Mg 2+ and K + ions, a series of mutants have been made and their activities were measured ( Fig. 4e ). These mutants and the EDTA-treated protein remain nearly as mono-disperse as the wild-type protein in solution ( Supplementary Fig. 9 ). When compared with the wild-type enzyme, the D249A and D219A mutants have lost 98.2% and 98.4% activity, respectively ( Fig. 4e ). The effect resembles that of EDTA to the wild-type enzyme activity because of the loss of Mg 2+ ion. Mutating either one of these two Asp residues to Ala will lead to dramatically reduced affinity of TmCdsA towards both Mg 2+ and K + ion, and thereby attenuates the enzyme activity. Asp249 is highly conserved among the prokaryotic and eukaryotic Cds homologues ( Supplementary Fig. 6 ). Although Asp219 is strictly conserved in the prokaryotic homologues ( Supplementary Fig. 6a ), it is often replaced by a Gly residue in the eukaryotic members ( Supplementary Fig. 6b ). The glycine residue may coordinate Mg 2+ ion directly through its carbonyl oxygen or indirectly through a nearby water molecule. In contrast to the strict conservation of Asp219 and Asp249 residues in prokaryotic Cds homologues, Glu222 is only partly conserved and is occasionally replaced by a Gln residue in Bacillus cereus or by a Lys residue in Aquifex aeolicus ( Supplementary Fig. 6a ). Curiously, the E222A mutant exhibits 16.7% of the wild-type activity ( Fig. 4e ), indicating a loss-of-function effect less severe than that of D249A or D219A mutation. As shown in Fig. 4d , Glu222 either directly interacts with K + ion through weak ionic bond or binds it indirectly through an unobserved water molecule inserted between them. Presumably, E222A mutation may lead to the loss or weakening of K + ion-binding site. Besides Asp219, Asp249 and Glu222 that are involved in Mg 2+ and K + binding, two additional acidic residues (Asp246 and Asp144) are found nearby the di-metal cofactor ( Fig. 4d ). These acidic residues form a patch of electro-negative surface that might represent a characteristic property of the Cds-active site ( Fig. 5c,d ). Binding of the two cations to the catalytic centre neutralizes the negative charges contributed by Asp219, Asp249 and Glu222. Moreover, Lys167 and Lys226 form ionic interactions with Asp219 and Asp246, respectively ( Fig. 4d ). Such interactions further neutralize the negative charges from the acidic residues on one hand and position the side chains of the key Asp residues properly within optimal region for catalysis on the other hand. Among the accessory charged residues, Lys167, Lys226, Asp144 and Asp246 are highly conserved among various prokaryotic and eukaryotic Cds proteins. Further mutagenesis analysis reveals that D144A, D246A, K226A and K167A mutants lost 98.5%, 99.7%, 98.8% and 99.2% of enzyme activity, respectively ( Fig. 4e ), indicating that they all have crucial roles in the function of TmCdsA. In comparison, the R166A mutant only loses 30.0% activity, consistent with the observation of Arg166 at a relatively distant location from the putative catalytic centre ( Fig. 4d ). From the structural view and verified by the point mutations described above, the active site of TmCdsA centres on the Mg 2+ -K + di-metal core coordinated by the Asp219-Asp249 dyad and also contains a series of accessory positively and negatively charged amino-acid residues that are crucial for the enzyme activity. 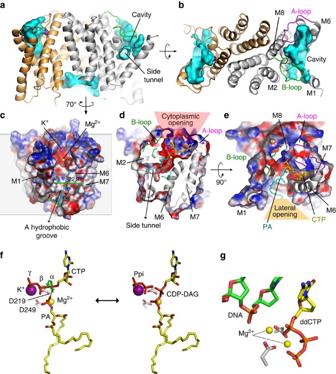Figure 5: The substrate binding cavity of TmCdsA and its catalytic mechanism. (a,b) The presence of two large cavities near the cytoplasmic surface of TmCdsA dimer. The cavities are shown as cyan surface models superposed on the cartoon representation of TmCdsA molecules. The front and top (from cytoplasmic side) views of TmCdsA dimer along the membrane plane and membrane normal are shown inaandb, respectively. (c) Side view of the electrostatic potential surface of TmCdsA. An elongated hydrophobic groove adjacent to the dual-opening cavity and exposed to the lipid bilayer is located on the outer surface of TmCdsA. The silver box shadow in the background indicates an estimated position of the membrane with respect to TmCdsA. The deep red and deep blue colours on the surfaces indicate electronegative and electropositive regions at −15 and 15 kT e−1, respectively. k, the Boltzmann constant; T, the temperature; e, the magnitude of the electron charge. The unit for the numbers above the dash lines is Å. (d) Sectional view of the funnel-shaped cavity within TmCdsA revealing an elongated side tunnel between the B-loop and M1 helix. The stick models of CTP (yellow) and PA (dioleoyl, cyan) are docked in the cavity through Autodock Vina programme51to show their predicted binding sites in TmCdsA. (e) The cavity viewed from the cytoplasmic side. For clarity, only the region surrounding the cavity is shown. (f) A proposed model for the catalytic mechanism of CDP-DAG synthesis. The green arrows indicate the nucleophilic attack on the α-phosphate of CTP launched by the Mg2+-activated PA head group and the withdrawing of electron, which leads to the break of α-β phosphodiester bond and production of pyrophosphate in addition to CDP-DAG. (g) The dual-Mg2+catalytic centre of human DNA polymerase in complex with both substrates, namely DNA and ddCTP (2′,3′-dideoxycytidine 5′-triphosphate). PDB code: 1BPY. Figure 5: The substrate binding cavity of TmCdsA and its catalytic mechanism. ( a , b ) The presence of two large cavities near the cytoplasmic surface of TmCdsA dimer. The cavities are shown as cyan surface models superposed on the cartoon representation of TmCdsA molecules. The front and top (from cytoplasmic side) views of TmCdsA dimer along the membrane plane and membrane normal are shown in a and b , respectively. ( c ) Side view of the electrostatic potential surface of TmCdsA. An elongated hydrophobic groove adjacent to the dual-opening cavity and exposed to the lipid bilayer is located on the outer surface of TmCdsA. The silver box shadow in the background indicates an estimated position of the membrane with respect to TmCdsA. The deep red and deep blue colours on the surfaces indicate electronegative and electropositive regions at −15 and 15 kT e −1 , respectively. k, the Boltzmann constant; T, the temperature; e, the magnitude of the electron charge. The unit for the numbers above the dash lines is Å. ( d ) Sectional view of the funnel-shaped cavity within TmCdsA revealing an elongated side tunnel between the B-loop and M1 helix. The stick models of CTP (yellow) and PA (dioleoyl, cyan) are docked in the cavity through Autodock Vina programme [51] to show their predicted binding sites in TmCdsA. ( e ) The cavity viewed from the cytoplasmic side. For clarity, only the region surrounding the cavity is shown. ( f ) A proposed model for the catalytic mechanism of CDP-DAG synthesis. The green arrows indicate the nucleophilic attack on the α-phosphate of CTP launched by the Mg 2+ -activated PA head group and the withdrawing of electron, which leads to the break of α-β phosphodiester bond and production of pyrophosphate in addition to CDP-DAG. ( g ) The dual-Mg 2+ catalytic centre of human DNA polymerase in complex with both substrates, namely DNA and ddCTP (2′,3′-dideoxycytidine 5′-triphosphate). PDB code: 1BPY. Full size image A funnel-shaped cavity with dual openings On the cytoplasmic side of each TmCdsA monomer, a funnel-shaped cavity embraces the di-metal core and indents half way into the membrane region ( Fig. 5a,b ). Its wall is mainly shaped by amino-acid residues from the CTD and NTD ( Fig. 5b ). Such an open cavity is reminiscent of the region for substrate binding. Recently, a different integral membrane enzyme named MraY, which is essential for bacterial cell wall synthesis, was reported to contain a U-shaped cavity predicted to be the binding site for its amphiphilic substrate molecule [33] . Although TmCdsA does not share any significant sequence homology or overall structural similarity with that of MraY, they both utilize dual substrates and require Mg 2+ ion for their activity. The cavity within TmCdsA has two wide openings, which enable it to receive dual substrates from cytoplasm and lipid bilayer at the same time ( Fig. 5c–e ). The opening facing cytoplasm ( Fig. 5d ) allows the water-soluble substrate, CTP/dCTP, to diffuse into the cavity and the by-product (pyrophosphate) to permeate back into cytosol. Meanwhile, the lateral opening ( Fig. 5e ) facilitates the hydrophobic substrate, namely PA, to access the cavity from the inner leaflet of lipid bilayer where it is synthesized [34] . After catalytic reaction, the lipophilic product, CDP-DAG, may also use the same lateral opening to return into the membrane region and serves as the substrate for further synthesis of various phospholipids. The relatively high B-factor of the M1 helix suggests a possibility that the lateral gate may be controlled by the pivoting movement of M1 helix against M2 helix. In this way, the access of PA molecule to the active site and the release of CDP-DAG can be regulated. Such an unusual funnel-shaped dual-opening cavity ( Fig. 5d ) is optimal for the integral membrane enzyme to perform catalysis on dual substrates with distinct property (one hydrophilic and the other hydrophobic) and release two products that also have different solubility in water/lipid. Substrate-dependent kinetic analysis results indicate that CTP binding exhibits positive cooperativity with an allosteric effect on TmCdsA, shown by the sigmoidal curve of the CTP-dependent kinetic (Hill coefficient=1.7, Supplementary Fig. 10a and Supplementary Table 1 ). In contrast, the PA-dependent kinetic data suggest there is little allosteric effect induced by PA binding (Hill coefficient=1.2, Supplementary Fig. 10b and Supplementary Table 1 ). Evidently, the affinity of TmCdsA for PA is higher than for CTP ( Supplementary Table 1 ). Earlier kinetic experiments on yeast Cds suggested that CTP binds to Cds before PA [20] , [35] . Which regions on TmCdsA are the potential binding sites for CTP and PA? As shown in Figure 5b,e , two cytoplasmic loops surround the active site and may exert their functional roles by contributing to substrate binding. They are the M6-M7 loop (A-loop) harbouring a conserved ‘SPXKXXEG’ motif and the M8-M9a loop (B-loop) covering a portion of the ‘HGGXXDRXD’ motif ( Supplementary Fig. 6a ). The A-loop forms close contacts with the C-terminal end of M8 helix ( Fig. 4d ), and along with M6 and M7 helices, they enclose a concave hydrophilic groove with a compatible physical shape for fitting the cytidine group of CTP, like a lock to the key ( Fig. 5e ). This area is most likely the basis for the enzyme to select CTP/dCTP instead of other nucleotides [18] . The S223C mutation on the C-terminal end of M8 helix has a dramatic effect on the enzyme activity ( Fig. 1c ), underscoring an important role of the interactions between the A-loop and M8 helix in Cds function. Meanwhile, the B-loop interacts with the N-terminal region of M1 helix. They enclose the central cavity from the opposite side of the A-loop and form an elongated side tunnel with half of its surface being hydrophilic and the other half hydrophobic ( Fig. 5d,e ). Such a special amphipathic tunnel tube is ideal for accommodating the glycerol-3-phosphate group of PA and one of its acyl chains ( Fig. 5d ). For the other acyl chain of PA molecule, a large hydrophobic groove (17–23 Å wide and ~24 Å long) located on the surface between the M1 and M7 helices is well-suited to provide its binding site and enrich the PA molecule from the membrane region ( Fig. 5c ). It was demonstrated earlier that the radioactivity of 32 P-labelled dipalmitoyl-PA can be transferred to the product molecule (CDP-DAG) by the Cds-catalysed reaction [9] , [36] . The enzymatic conversion of CTP and PA into CDP-DAG and pyrophosphate occurs through a process involving the transfer of cytidyl-monophosphatidyl group from CTP onto the phosphate group of PA. In the past nearly five decades since Carter and Kennedy first reported enzymatic synthesis of CDP-DAG in 1966 (ref. 15 ), the mechanistic details of this fundamental process have remained poorly defined due to the lack of structural information of the Cds family. Now, with the crystal structure of TmCdsA being solved, it becomes possible to deduce the catalytic mechanism of Cds by comparing its active site structure to those of other nucleotidyltransferases such as the DNA polymerases. As shown in Fig. 5g , the DNA polymerases use a two-metal-ion centre (dual Mg 2+ ions named metals A and B) to catalyse the transfer of the nucleotidyl-monophosphatidyl group of dNTP onto the 3′-hydroxyl group of a DNA molecule [37] , [38] . The two-Mg 2+ -ion catalysis is widely used by nucleic acid enzymes including nucleases and transposases besides the DNA/RNA polymerase [39] , [40] . By analogy, the Cds may adopt a catalytic process, which involves breaking of the α-β phosphodiester bond of the nucleotide molecule and subsequent transferring of the cytidyl-monophosphatidyl group to PA molecule. The Mg 2+ ion in TmCdsA might serve as the metal A that is responsible for activating the phosphate group of PA molecule and promotes its nucleophilic attack on the α-phosphate of CTP ( Fig. 5f ), whereas the K + ion likely serves as the metal B that binds to the β- and γ-phosphates of CTP and facilitates the dissociation of pyrophosphate from the active site. Thereby, TmCdsA represents a unique integral membrane enzyme discovered to contain a non-canonical Mg 2+ -K + hetero-di-metal centre for its catalytic function. As for the accessory charged amino-acid residues around the active site, such as Asp144, Lys167, Lys226 and Asp 246, which are shown to be crucial for the enzyme activity ( Fig. 4e ), they may contribute to the catalytic process by binding to the polar groups of substrate molecules, facilitating the formation of intermediate product or assisting with the dissociation of the final products from the active site. Protein expression and purification The gene encoding a CdsA homologue was amplified from the genomic DNA of T. maritima using the following pair of primers: forward primer: 5′-CGGCAGCCATATGGATGATTTGAAAACCAGAG-3′ and reverse primer: 5′-TCCGGATCCTCATCGCACCACTCCTTCTAAG-3′. The gel-purified DNA was digested and then ligated into the pET15b vector between Nde I and Bam HI sites. The plasmid was transformed into C41(DE3) E. coli strain. For protein expression, every 2-l Terrific Broth media in a 5-l baffled flask was inoculated with 50 ml overnight culture seeded from a single colony on a LB-Amp plate or from a tube of defrosted glycerol stock culture stored at −80 °C. When the cell density reached 1.0 OD 600 nm , the inducer isopropyl-β- D -thiogalactoside was added to the culture to a final concentration of 0.5 mM. The protein expression continued for 2 h at 37 °C before the cells were harvested by centrifugation at 6,000 r.p.m. and then stored at −80 °C. The frozen cell pellets were suspended in lysis buffer (50 mM Tris–HCl, 300 mM NaCl, pH 8.0) at 0.1 g ml −1 ratio and then homogenized by T10 basic homogenizer (IKA). To lyse the cell and extract membrane proteins, 1.5 g decyl-β- D -maltoside (DM; Anatrace) powder was added to 100 ml cell suspension, which was subsequently stirred on ice to dissolve the detergent powder completely and then sonicated with Misonic sonicator 4000 programmed at 80% power with the setting of 1 s on (for 2 min total) and 5 s off. After sonication, the cell lysate turned semi-transparent and was subject to centrifugation at 17,000 r.p.m. in JA-25.50 rotor (Beckman) for 40 min to remove insoluble debris. The supernatant was loaded slowly onto a gravity column with 1 ml Ni-NTA resin per 50 ml supernatant. The column was pre-equilibrated by five volumes of buffer A (25 mM Tris–HCl, 300 mM NaCl, 20 mM imidazole, 0.5% DM, pH 7.5). After the sample flowed through, the resin was washed with five column volumes of buffer A and then five volumes of buffer B (25 mM Tris–HCl, 300 mM NaCl, 70 mM imidazole, 0.4% DM, pH 7.5). The target protein was eluted with buffer C (25 mM Tris-HCl, 300 mM NaCl, 300 mM imidazole, 0.3% DM, pH 7.5). The fractions with protein concentration greater than 0.5 mg ml −1 were combined and immediately diluted by two volumes of buffer D (10 mM Tris–HCl, 300 mM NaCl, 50 mM MgCl 2 , 0.3% DM, pH 7.5) to prevent the protein from precipitating. After being concentrated to ~15 mg ml −1 in 50 kDa concentrator (Millipore), the protein sample was loaded onto Superdex 200 10/300 GL column (GE Healthcare) and eluted in buffer E (10 mM Tris-HCl, 300 mM NaCl, 50 mM MgCl 2 , 0.4% nonyl-β- D -glucoside (NG), pH 7.5). The fractions between 11.6 and 13.6 ml were pooled and concentrated to 20 mg ml −1 for crystallization experiments. For enzyme activity assays on the wild-type and mutant proteins, the gel filtration step was skipped. Instead of using DM, n -dodecyl-β- D -maltoside (DDM, Anatrace) was used in buffer A-C (0.1% DDM in buffer A and 0.05% DDM in buffer B and C). The protein sample eluted from Ni-NTA column was exchanged into an imidazole-free buffer (25 mM Tris-HCl, 500 mM NaCl, 2 mM DTT, 20% glycerol, 0.05% DDM, pH 7.5) within the concentrator. To prepare the salt-free protein sample for the test of activity-stimulating effect of cations shown in Fig. 4a,b , the protein was dialysed extensively against a dialysis buffer containing no salt (25 mM Tris–HCl, 20% glycerol, 2 mM DTT, 0.05% DDM, pH 7.5). Crystallization and heavy-atom derivative preparation For the growth of hexagonal rod crystals in P6 5 22 space group, 10 μl of 20 mg ml −1 S200C/S223C mutant protein was mixed with 1.1 μl 20 mM CH 3 HgCl, and then centrifuged at 14,000 r.p.m. for 10 min to remove pellets. The hanging drops were set up by combining 1.0 μl of protein-CH 3 HgCl mixture with 1.0 μl of well solution (8–13% PEG3350, 100 mM NaCl, 20 mM HEPES, pH 7.0) and then equilibrated against 200 μl well solution at 16 °C. Hexagonal rod crystals usually appear within 2 days and mature to 0.2–0.3 mm in length in about 1 week. For S33C or A62C mutants ( Supplementary Fig. 3d ), monoclinic crystals of C2 space group were grown under similar condition (well solution: 9–13% PEG3350, 100 mM NaCl, 20 mM HEPES, pH7.0) when there is no CH 3 HgCl added to the protein sample before crystallization. The mercury was introduced by soaking the crystals in a derivatizing solution containing 1 mM CH 3 HgCl, 12% PEG3350, 100 mM NaCl, 20 mM HEPES, pH 7.0. For the preparation of Ba 2+ -containing sample, the S200C/S223C crystal was soaked overnight in a solution with 50 mM BaCl 2 , 100 mM NaCl, 12% PEG3350, 0.4% NG and 20 mM HEPES, pH 7.0. The Mn 2+ -containing crystal was prepared by soaking in a solution with 10 mM MnCl 2 , 100 mM KCl, 12% PEG3350, 0.4% NG and 20 mM HEPES, pH 7.0 for 8 h. As for the Tl + /Cs + -containing crystals, they were prepared by soaking overnight in a solution (containing 25 mM MgCl 2 ) with 100 mM TlNO 3 or 300 mM CsCl instead of KCl/NaCl. For obtaining the crystals with both Rb + and Mn 2+ , they were soaked for 1.5 h in a solution with 200 mM RbCl and 10 mM MnCl 2 . The crystals were cryoprotected with 15% glycerol through a step-wise transfer procedure and then flash-frozen by dunking into liquid N 2 . The high-quality S200C/S223C crystal used for the collection of 3.4 Å-resolution data was prepared by soaking it in a solution with 100 mM KCl, 25 mM MgCl 2 , 11% PEG3350, 0.4% NG, 20 mM HEPES (pH 7.0) and 15% glycerol. The S200C/S258C (active mutant) crystal was briefly soaked in 100 mM NaCl, 14% PEG3350, 0.4% NG, 20 mM HEPES (PH7.0) and 15% glycerol before being frozen and used for data collection. Data collection and processing Crystal screening and diffraction quality evaluation was mainly carried out at the in-house X-ray source and the BL17U beamline of Shanghai Synchrotron Radiation Facility (SSRF). The data set used for phasing was collected at the BL5A of Photon Factory (PF, Tsukuba, Japan) with ADSC Q315 CCD detector. The anomalous diffraction data sets of site-directed cysteine mutant crystals labelled with mercury for the verification of sequence registration on the structural model were collected on SSRF BL17U and PF BL5A/NE3A. A high-quality data set of S200C/S223C crystal used for the final structure refinement was collected at the BL1A micro-focus beamline of PF with PILATUS 2M-F detector. To minimize radiation damage, the ‘helix mode’ was applied for data collection of a total of 60° oscillation range (1°/frame) on three individual spots on the crystal to yield a complete data set. The data set of S200C/S258C mutant crystal was collected at SSRF BL17U beamline with ADSC Q315r detector. The data of BaCl 2 , MnCl 2 , TlNO 3 , CsCl or MnCl 2 +RbCl-soaked crystals were all collected with the in-house Rigaku MicroMax-007 rotating anode X-ray generator and Raxis IV detector. All data sets were collected under 100 K condition. The HKL2000 (ref. 41 ) or iMOSFLM [42] programmes were used for data processing. Structure determination and analyses To solve the phases of structure factors, the high-redundancy data set of S200C/S223C crystal ( Table 1 ) with Hg anomalous signals was input to the Phenix [43] Autosol programme for the search of six heavy atom sites. Density modification was run automatically in the Phenix suite after the initial single-wavelength anomalous dispersion phases were obtained. The figure of merit increased from 0.34 to 0.60 after density modification. A partial structural model was built through Phenix Autobuild ( Supplementary Fig. 3a,b ). The model was corrected and completed gradually through iterative refinement and rebuilding cycles guided by the 11 site-specific mercury labels shown in Supplementary Fig. 3c,d , and the improved 2 F o − F c maps obtained through density modification (including solvent flattening and twofold NCS averaging) by using the DM programme in CCP4 suite [44] . The Coot programme [45] was used for model building and visualizing the electron density maps/structures. The structures were refined by the CNS 1.2 programme [46] with maximum likelihood target function using amplitudes. The final model phases have figure of merit values at 0.695 or 0.744 for the S200C/S223C or S200C/S258C structures. The 2 F o − F c map at 3.4 Å resolution exhibited features matching well with the model in most regions including the transmembrane helices and loops ( Fig. 2 ). Procheck [47] was used to analyse the quality and geometry of the structural models. Ramachandran plot statistics of the S200C/S223C (or S200C/S258C) structures are 92.7% (or 90.1%), 6.9% (or 9.9%) and 0.4% (or 0.0%) for the most favoured, additional allowed and generously allowed regions, respectively. No residues are in the disallowed region in both structures. For the detection of helix kinks, the HELANAL programme [48] was used. The cartoon structural models were generated through Pymol [49] programme. The PRALINE TM programme with an algorithm optimized for transmembrane protein sequence alignment [50] was used for the alignment of multiple Cds homologues. AutoDock Vina programme [51] was used to search for potential binding sites of substrate molecules (namely, CTP and dioleoyl phosphatidic acid (DOPA)) within TmCdsA. The CTP molecule was docked first and then merged with the protein structure. The combined coordinate data were subsequently input to AutoDock Vina again to perform a second-round search for DOPA-binding site. The phosphate groups of CTP and DOPA were manually adjusted through torsion around rotatable bonds to adopt the estimated optimal positions for reaction. Activity assay with radioactive labelled substrate The assay method for measuring TmCdsA enzyme activity was adapted from the protocols described in refs 18 , 52 . The [5- 3 H]-CTP (specific activity at 18.8 or 20 Ci mmol −1 , PerkinElmer or American Radiolabeled Chemicals) was used as the radiolabelled substrate for the detection of liponucleotide product. In brief, a 50-μl reaction contains 4 mM [5- 3 H]-CTP (specific activity at 10 Ci mol −1 ), 2 mM DOPA (Avanti Polar Lipids), 2 mM MgCl 2 (Sigma), 50 mM Tris–HCl (pH7.5; Amresco), 0.25 mM DTT (Merck), 200 mM KCl (Sigma), 1 mg ml −1 bovine serum albumin (Amresco), 10 mM Triton X-100 (Sigma) and enzyme. The velocity of the reaction catalysed by wild-type TmCdsA was linear within 60 min at 30 °C. For the data shown in Fig. 1c , the reactions except the control (no enzyme added) were performed with 80.6 ng enzyme (at 50 nM concentration) for 30 min, whereas for those shown in Fig. 4e and Supplementary Fig. 10 , 30 ng enzyme and 10 min reaction time were used. After reaction, 180 μl of chloroform/methanol/concentrated HCl (1:2:0.02, v/v/v) mixture was added to the tube, followed by further addition of 60 μl of chloroform and 60 μl of 2 M KCl per tube. The tubes were vortexed and then centrifuged for 15 min at 5,000 r.p.m. to separate the organic phase from the aqueous phase. For the measurement of product radioactivity, every 40 μl of the lower organic phase was mixed with 1 ml OptiPhase Supermix Cocktail scintillation liquid (PerkinElmer). After thorough mixing by vigorous vortexing, the sample was subjected to liquid scintillation counting in the Wallac 1,450 MicroBeta trilux liquid scintillation and luminescence counter (PerkinElmer). Three or four parallel repeat experiments were performed for the measurement of each data point. For the CTP- or PA-dependent kinetic assays, wild-type TmCdsA enzyme was used and the concentration of DOPA/CTP was held constant at 2 mM/4 mM, whereas the concentration of the other one was varied from 0.05 to 5 or 0.05 to 2 mM as shown. GraphPad Prism programme was used for fitting the substrate-dependent kinetic data. To analyse the Mg 2+ -dependent or monovalent cation- (all cations were added in the form of chloride salts) dependent behaviours, the reactions were performed with 2 μM enzyme, 2 mM [5- 3 H]-CTP (with specific activity at 1.88 Ci mol −1 ) and 1 mM DOPA for 10 min. Crosslinking and light-scattering experiments For the crosslinking experiments, 10 μg purified TmCdsA, S200C/S223C, S200C/S258C protein were added to 10 μl reaction systems with 20 mM HEPES (pH 7.5), 100 mM NaCl and 0.3% β-DM. The crosslinker glutaraldehyde (Sigma) was added into the reaction systems to the final concentrations at 0, 3.3 or 10 mM. The reaction was carried out at 25 °C for 30 min and stopped by adding Tris–HCl buffer (pH7.5) to 100 mM concentration. Aliquots of 10 μl reaction solution were analysed by SDS–polyacrylamide gel electrophoresis. For the time-dependent crosslinking experiments, 100 mM stock solution of glutaraldehyde was added into the reaction system to a final concentration at 10 mM. Aliquots of reaction products were sampled at 0, 20 and 240 min, respectively, quenched and then used for SDS–polyacrylamide gel electrophoresis analysis. For the measurements of oligomeric state/protein masses of TmCdsA in solution, the size-exclusion chromatography coupled with multi-angle light scattering (SEC-MALS) method was applied. The system consists of a 1200 series HPLC system (Agilent Technologies), a DAWN HELEOS-II instrument (Wyatt) and an Optilab rEX refractive index instrument (Wyatt). To apply the samples, 50 μl of wild-type, S200C/S223C or S200C/S258C TmCdsA protein samples purified in DM (protein concentration at around 4 mg ml −1 ) were injected into the WTC-030S5 SEC column (Wyatt) and eluted at 0.5 ml min −1 in a buffer containing 10 mM Tris-HCl, 300 mM NaCl, 50 mM MgCl 2 , 0.3% DM, pH 7.5. The extinction coefficient of protein at 280 nm was calculated from the amino-acid sequences ( A 280 (wild type)=0.771 ml mg −1 cm −1 , A 280 (S200C/S223C)=0.770 ml mg −1 cm −1 , A 280 (S200C/S258C)=0.770 ml mg −1 cm −1 ). The detergent DM has no absorbance at 280 nm. Data collection and analysis were performed with Astra 5 software (Wyatt). The specific refractive index ( dn/dc ) value of protein (TmCdsA, S200C/S223C and S200C/S258C) at 0.185 ml g −1 and that of DM at 0.1473, ml g −1 were used for data processing. The total molecular masses and individual masses of the proteins and the detergent were determined with Astra 5 software using protein conjugate analysis. The peak overlap and peak broadening corrections were carried out with Astra 5 software. The SEC-MALS system was pre-calibrated with bovine serum albumin protein standard. To analyse the mono-dispersity of protein samples used for activity assays, the protein samples were run through Superdex 200 10/300 GL gel filtration column in a buffer with 50 mM Tris-HCl (pH 7.5), 0.25 mM DTT, 200 mM KCl, 2 mM MgCl 2 and 0.05% DDM (for the EDTA-treated protein, the MgCl 2 was replaced by 5 mM EDTA). The main peak at around 12.8 ml was collected and subject to dynamic light-scattering (DLS) analysis using the DynaPro NanoStar instrument (Wyatt). The DLS measurements were performed at 25 °C using 10 μl gel-filtration purified protein samples (0.2 mg ml −1 ) and the averaged data of ten readings (5 s each) were recorded. The DLS data were analysed with DYNAMICS V7.0 programme. Accession codes: Atomic coordinates and structure factors for TmCdsA have been deposited in the Protein Data Bank under accession codes 4Q2E (S200C/S223C) and 4Q2G (S200C/S258C). How to cite this article: Liu, X. et al . Structure and mechanism of an intramembrane liponucleotide synthetase central for phospholipid biosynthesis. Nat. Commun. 5:4244 doi: 10.1038/ncomms5244 (2014).